Integrin β1 controls VE-cadherin localization and blood vessel stability Angiogenic blood vessel growth requires several distinct but integrated cellular activities. Endothelial cell sprouting and proliferation lead to the expansion of the vasculature and give rise to a highly branched, immature plexus, which is subsequently reorganized into a mature and stable network. Although it is known that integrin-mediated cell–matrix interactions are indispensable for embryonic angiogenesis, little is known about the function of integrins in different steps of vascular morphogenesis. Here, by investigating the integrin β1-subunit with inducible and endothelial-specific gene targeting in the postnatal mouse retina, we show that β1 integrin promotes endothelial sprouting but is a negative regulator of proliferation. In maturing vessels, integrin β1 is indispensable for proper localization of VE-cadherin and thereby cell–cell junction integrity. The sum of our findings establishes that integrin β1 has critical functions in the growing and maturing vasculature, and is required for the formation of stable, non-leaky blood vessels. The vasculature has essential functions in the healthy organism and defects affecting the integrity or angiogenic growth of blood vessel are associated with a wide range of pathobiological processes [1] , [2] , [3] . Depending on disease characteristics and patient needs, it can be desirable to form new blood vessels, for example, to promote wound healing and regeneration, whereas anti-angiogenic therapies have been already used to inhibit pathological neovascularization or suppress harmful vessel leakage. Integrin family receptors and associated components of the cell–matrix adhesion machinery, such as focal adhesion kinase (FAK), integrin-linked kinase, kindlin or talin are also recognized key regulators of endothelial cell function and angiogenesis [4] , [5] , [6] , [7] . Integrins, which are heterodimeric receptors formed by transmembranous α- and β-subunits, can bind a wide range of different extracellular matrix (ECM) proteins, as well as certain soluble factors and cell surface proteins. In addition to outside-in signalling, which involves substrate binding, integrin activation and downstream signal transduction, changes in integrin conformation can be induced by intracellular triggers such as talin/kindlin binding or activity of the small GTPase Rap1, a process termed inside-out activation [8] , [9] , [10] . In the vasculature, the integrins αvβ3 and αvβ5 have been linked to angiogenesis and the activation of vascular endothelial growth factor (VEGF) receptors [1] , [11] . The β1-subunit, which can partner with 12 different α-chains and plays a central role in cell–matrix adhesion, has been also investigated with EC-specific gene targeting approaches in mice. Constitutive targeting of Itgb1 , the gene encoding integrin β1, in ECs was found to be incompatible with normal morphogenesis of the embryonic vasculature and survival beyond midgestation [12] , [13] , [14] . Although this work has established that endothelial Itgb1 gene function is required for angiogenic sprouting but not for the assembly of the first vessel primordia by vasculogenesis, insight into the precise function of integrin β1 in the regulation of angiogenesis was limited by early embryonic lethality. More recently, tamoxifen-inducible mutants were generated and, based on the occurrence of occlusions that were exclusively observed in arteries, it was proposed that integrin β1 controls arteriolar lumen formation [15] . The normal appearance of other vessel beds in these mutants suggested surprisingly limited roles of β1-containing integrins in angiogenesis. Here we have reinvestigated the role of the β1-subunit in an independent approach using different conditional Itgb1 allele [16] and tamoxifen-inducible Cre strains [17] . We have focused on the postnatal vascularization of the retina, which allows high-resolution imaging and has hugely advanced the characterization of angiogenesis in the mouse model [18] , [19] . This approach has uncovered novel and critical roles of integrin β1 in the growing vasculature. Our findings also link the β1-subunit and thereby cell–matrix interactions to the regulation of junctional integrity, which has important implications for pathobiological conditions with increased vascular permeability. Inducible inactivation of Itgb1 in the postnatal endothelium The integrin β1-subunit is prominently expressed in the postnatal retinal vasculature. In particular, strong antibody staining was seen in arteries, capillaries and veins, in vascular smooth muscle cells, throughout the newly formed vessel plexus at the angiogenic growth front, and in distal endothelial sprouts ( Supplementary Fig. 1 ). Very similar staining patterns were obtained with an antibody recognizing the active conformation of integrin β1 (ref. 20 ; Supplementary Fig. 2a,b ). The analysis of different postnatal stages between postnatal day (P) 6 and P60 revealed that active integrin β1 immunosignals were notably higher in the remodelling and maturing endothelium (that is, from P10 onwards) than in the actively growing retinal vasculature at P6 ( Supplementary Fig. 2c ). To inactivate Itgb1 in postnatal ECs, mice carrying a loxP-flanked allele of the gene [16] were bred to tamoxifen-inducible Pdgfb-iCre transgenics [17] . Tamoxifen administration and induction of Itgb1 inactivation at different stages impaired the health, mobility and, finally, survival of Pdgfb-iCre+ , Itgb1 lox/lox ( Itgb1 iECKO ) mutants. As tamoxifen-treated control littermates were not affected, these phenotypes were caused by the loss of integrin β1 in ECs and, consequently, animals were killed and analysed at humane endpoints ( Supplementary Fig. 3a ). In line with the limited survival of Itgb1 iECKO mutants, vascularization of the retina was impaired and vascular integrin β1 staining was strongly decreased ( Supplementary Fig. 3b–e ). This established that the inducible strategy enabled rapid and reliable inactivation of Itgb1 in the postnatal vasculature. Characterization of the vascular defects in P6 Itgb1 iECKO retinas showed that radial vessel outgrowth and endothelial sprouting were strongly compromised ( Fig. 1a–e and Supplementary Fig. 3b ). Although mutant ECs at the leading edge extended bursts of filopodia that were even longer and more abundant than in controls, sprouts failed to extend and the distal edge of the vascular plexus appeared blunt ( Fig. 1a–d ). Similar sprouting defects were observed in P9 Itgb1 iECKO retinas and, at the same time, the peripheral vascular plexus was strongly condensed so that individual vessels were no longer distinguishable ( Fig. 1a and Supplementary Fig. 4a,b ). Despite the strongly compromised sprouting and radial outgrowth, expression of Esm1, a tip cell marker that is induced by VEGF-A [21] , [22] , was maintained in a fraction of EC at the angiogenic growth front ( Supplementary Fig. 4c ). This suggested that integrin β1 is not required for signalling processes leading to the induction of potential tip cells, but is indispensable for the extension of endothelial sprouts. This role was not confined to the extension of the superficial vessel plexus and vascularization of the deeper Itgb1 iECKO retina was strongly compromised at P9 ( Supplementary Fig. 4d ). Furthermore, we confirmed that the dense appearance of the distal vasculature in mutant retinas ( Fig. 1a ) was caused by endothelial cell hyperproliferation. Labelling of mitotic cells by incorporation of EdU showed strongly increased proliferation of integrin β1-deficient ECs, which was most prominent in the distal perivenous vessel plexus ( Supplementary Fig. 4a,b ). Protein levels of p27Kip1, a cell cycle inhibitor, and of cyclin D1, a cell cycle regulator that is low in S-phase, were substantially reduced in Itgb1 iECKO lung lysates ( Supplementary Fig. 4e ). 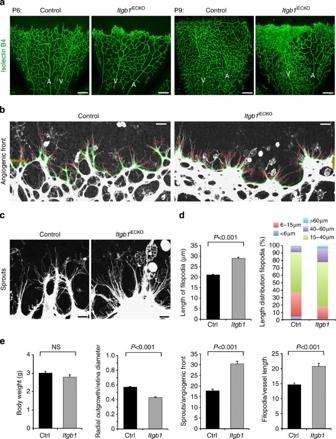Figure 1: Integrin β1 is indispensable for sprout formation. (a) Maximum intensity projection of confocal images showing the control andItgb1iECKOmutant retinal vasculature P6 and P9, respectively. Veins (V) and arteries (A) are indicated. The density of mutant vessels was increased at the angiogenic front, but decreased around arteries. ECs, isolectin B4 (green). Scale bar, 200 μm. (b) Appearance of the P6 control andItgb1iECKOvessel growth front and quantitative analysis of filopodia (red marks) per vessel length (green). Scale bar, 25 μm. (c) High-magnification confocal images of filopodia-extending cells at the edge of the control and mutant angiogenic growth front. Note the absence of extending sprouts despite the presence of filopodial bursts in the P6Itgb1iECKOvasculature. Scale bar, 10 μm. (d,e) Quantitation of body weight, radial outgrowth of the retinal vasculature, as well as ratios of the number of filopodia bursts (sprouts) or individual filopodia divided by the length of the vascular front (green line inb). Average length and length distribution of filopodial protrusions were shown ind. Error bars, s.e.m.P-values, Student’st-test (n=4 mice per group). NS, not statistically significant. Figure 1: Integrin β1 is indispensable for sprout formation. ( a ) Maximum intensity projection of confocal images showing the control and Itgb1 iECKO mutant retinal vasculature P6 and P9, respectively. Veins (V) and arteries (A) are indicated. The density of mutant vessels was increased at the angiogenic front, but decreased around arteries. ECs, isolectin B4 (green). Scale bar, 200 μm. ( b ) Appearance of the P6 control and Itgb1 iECKO vessel growth front and quantitative analysis of filopodia (red marks) per vessel length (green). Scale bar, 25 μm. ( c ) High-magnification confocal images of filopodia-extending cells at the edge of the control and mutant angiogenic growth front. Note the absence of extending sprouts despite the presence of filopodial bursts in the P6 Itgb1 iECKO vasculature. Scale bar, 10 μm. ( d , e ) Quantitation of body weight, radial outgrowth of the retinal vasculature, as well as ratios of the number of filopodia bursts (sprouts) or individual filopodia divided by the length of the vascular front (green line in b ). Average length and length distribution of filopodial protrusions were shown in d . Error bars, s.e.m. P -values, Student’s t -test ( n =4 mice per group). NS, not statistically significant. Full size image Matrix deposition and vessel stability in Itgb1 mutants Consistent with the role of integrins as cell–matrix receptors, ECM deposition was altered in the P6 Itgb1 iECKO retinal vasculature. Antibody signals for laminin α4 were enhanced, whereas anti-fibronectin signals were decreased ( Supplementary Fig. 5a,b ). Quantitative PCR showed elevated expression of messenger RNA encoding Mmp9, a matrix metalloproteinase that degrades fibronectin and other matrix molecules, in Itgb1 iECKO lung lysate. In contrast, Mmp2 and Mmp14 transcripts were not changed significantly ( Supplementary Fig. 5c ). The same analysis also revealed a small but significant decrease in expression of Kdr / Vegfr2 , the receptor for VEGF-A ( Supplementary Fig. 5c ). Transmission electron microscopy showed a strong reduction of the subendothelial basement membrane in Itgb1 mutant vessels, whereas no such decrease was seen for the ECM ensheating the outer surface of pericytes ( Supplementary Fig. 5d ). These data indicate that endothelial integrin β1 controls vascular ECM deposition and proper organization of the vessel wall. The characterization of Itgb1 iECKO mutants also uncovered a critical role of the β1-subunit in vessel stability. Pruning of capillaries around developing arteries was increased, leading to a significant reduction of arterial branch points ( Fig. 2a–c ). In contrast, density and branching of the Itgb1 iECKO perivenous vessel plexus was significantly increased ( Fig. 2a–c ). Although few endothelial sprouts were seen in the P9 control perivenous plexus, ectopic filopodia-extending cells were abundant in the equivalent region of the mutant vasculature ( Fig. 2d ). Empty collagen IV+, isolectin B4- matrix sleeves and well-established indicators of vessel retraction [23] were highly abundant in the Itgb1 iECKO vasculature ( Fig. 2e ). Thus, although β1 is required for endothelial sprouting at the vessel growth front and into the deeper retina, the subunit is also indispensable for the formation of stable and mature vessels, and suppresses angiogenic activities such as proliferation and sprouting in a context-dependent manner. 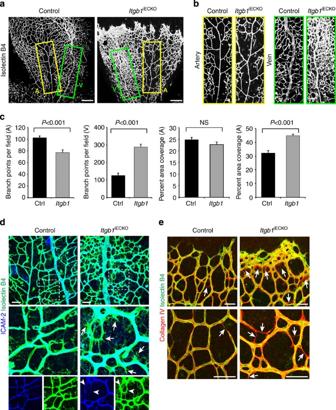Figure 2: Destabilization ofItgb1mutant retinal vessels. (a,b) Confocal images showing isolectin B4-stained P9 retina whole mounts. Higher magnification of periarterial (A, yellow frames) and perivenous (V, green frames) regions are displayed inb. Note enlarged capillary-free area aroundItgb1iECKOarteries, but higher vessel density around mutant veins relative to control littermate samples. Scale bar, 200 μm. (c) Quantitation of branch points and vessel-covered areas around arteries (A) and veins (V). Error bars, s.e.m.P-values, Student’st-test (n=4 mice per group). NS, not statistically significant. (d) Maximum intensity projection of perivenous blood vessels in the P6 central retina stained with isolectin B4 (green) and, for the visualization of vessel lumens, anti-ICAM2 antibody (blue). Note abundance of ectopic sprouts (arrows) inItgb1iECKOmutants, which was accompanied by loss of apical ICAM2 signal (arrowheads). Scale bar, 50 μm. (e) Representative images showing increased occurrence of empty collagen IV+ (red) but isolectin B4 (green)-negative matrix sleeves (arrows) at the P6Itgb1iECKOangiogenic front (top) and in vessels of the central retina (bottom). Scale bar, 50 μm. Figure 2: Destabilization of Itgb1 mutant retinal vessels. ( a , b ) Confocal images showing isolectin B4-stained P9 retina whole mounts. Higher magnification of periarterial (A, yellow frames) and perivenous (V, green frames) regions are displayed in b . Note enlarged capillary-free area around Itgb1 iECKO arteries, but higher vessel density around mutant veins relative to control littermate samples. Scale bar, 200 μm. ( c ) Quantitation of branch points and vessel-covered areas around arteries (A) and veins (V). Error bars, s.e.m. P -values, Student’s t -test ( n =4 mice per group). NS, not statistically significant. ( d ) Maximum intensity projection of perivenous blood vessels in the P6 central retina stained with isolectin B4 (green) and, for the visualization of vessel lumens, anti-ICAM2 antibody (blue). Note abundance of ectopic sprouts (arrows) in Itgb1 iECKO mutants, which was accompanied by loss of apical ICAM2 signal (arrowheads). Scale bar, 50 μm. ( e ) Representative images showing increased occurrence of empty collagen IV+ (red) but isolectin B4 (green)-negative matrix sleeves (arrows) at the P6 Itgb1 iECKO angiogenic front (top) and in vessels of the central retina (bottom). Scale bar, 50 μm. Full size image Integrin β1 controls junctional integrity Previous work has established that VE-cadherin, a main component of endothelial adherens junctions, is essential for angiogenesis and, in particular, the suppression of EC sprouting and proliferation [24] , [25] . We found that VE-cadherin distribution was substantially altered in Itgb1 iECKO retinal vessels ( Fig. 3a ). Although the adhesion protein decorated cell–cell junctions and showed strong overlap with Claudin 5 in the P9 control vasculature, VE-cadherin was found in punctate clusters and its junctional distribution was discontinuous in the Itgb1 iECKO endothelium ( Fig. 3a ). Furthermore, ultrastructural analysis confirmed junctional defects in Itgb1 mutant retinal vessels, which included discontinuous distribution of electron-dense protein complexes or the appearance of cyst-like structures at cell–cell contact sites ( Fig. 3b ). Junction defects were observed in Itgb1 iECKO mutants at different postnatal stages and affected mainly veins and perivenous capillaries, whereas arterial anti-VE-cadherin immunostaining appeared comparable to control littermates ( Supplementary Figs 6a,b and 7 ). 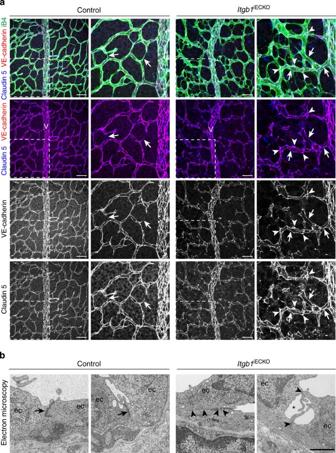Figure 3: Junctional defects in theItgb1endothelium. (a) Confocal images of isolectin B4 (green)-, anti-Claudin 5 (blue)- and anti-VE-cadherin (red)-stained capillaries surrounding veins (V) in the P9 retina, as indicated. Single channels are shown in rows 3 and 4. Spot-like VE-cadherin clusters (arrowheads) and EC–EC contacts with weak or absent VE-cadherin signal (arrows) were abundant inthe Itgb1iECKOendothelium. Scale bar, 50 μm. (b) Electron micrographs showing continuous, electron-dense junctions in P18 control retinal vessels (arrows). Targeting ofItgb1from P10 onwards led to discontinuous junctional contacts (arrowheads) and the appearance of cyst-like structures (asterisk) between endothelial cells (ec). Scale bar, 1 μm. Figure 3: Junctional defects in the Itgb1 endothelium. ( a ) Confocal images of isolectin B4 (green)-, anti-Claudin 5 (blue)- and anti-VE-cadherin (red)-stained capillaries surrounding veins (V) in the P9 retina, as indicated. Single channels are shown in rows 3 and 4. Spot-like VE-cadherin clusters (arrowheads) and EC–EC contacts with weak or absent VE-cadherin signal (arrows) were abundant in the Itgb1 iECKO endothelium. Scale bar, 50 μm. ( b ) Electron micrographs showing continuous, electron-dense junctions in P18 control retinal vessels (arrows). Targeting of Itgb1 from P10 onwards led to discontinuous junctional contacts (arrowheads) and the appearance of cyst-like structures (asterisk) between endothelial cells (ec). Scale bar, 1 μm. Full size image In line with the defective organization of Itgb1 iECKO junctions, extensive haemorrhaging was observed in freshly isolated mutant retinas ( Fig. 4a ). Confocal microscopy further confirmed the extravasation of Ter-119+ red blood cells in Itgb1 iECKO but not control animals ( Fig. 4b ). These defects were not confined to the retina and signs of focal haemorrhaging and perivascular accumulation of extravasated red blood cells were also seen in Itgb1 iECKO mutant brains ( Fig. 4c–e ). 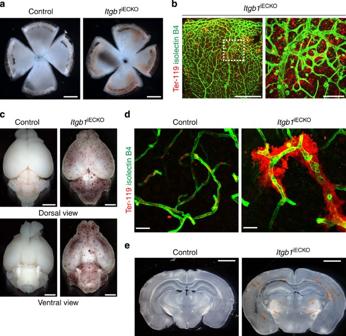Figure 4: Loss of vascular integrity in EC-specificItgb1mutants. (a) Haemorrhaging was evident in freshly dissectedItgb1iECKOP9 retinas but not in littermate control samples. Scale bar, 500 μm. (b) Ter-119-positive erythrocytes (red) in P18Itgb1iECKOretinal tissue outside the vasculature. Image in the right shows higher magnification of inset. ECs, isolectin B4 (green). Scale bar, left, 500 μm, right, 100 μm. (c) Haemorrhaging in freshly dissectedItgb1iECKOP9 brains affecting the cortex, cerebellum, brain stem and the olfactory bulbs. Scale bar, 2 mm. (d) Anti-Ter-119 (red) and isolectin B4 (green) immunofluorescence showing strong accumulation of red blood cells aroundItgb1iECKObrain capillaries. Scale bar, 25 μm. (e) Sections of P18 control andItgb1iECKObrains showing prominent haemorrhaging in mutants. Scale bar, 2 mm. Figure 4: Loss of vascular integrity in EC-specific Itgb1 mutants. ( a ) Haemorrhaging was evident in freshly dissected Itgb1 iECKO P9 retinas but not in littermate control samples. Scale bar, 500 μm. ( b ) Ter-119-positive erythrocytes (red) in P18 Itgb1 iECKO retinal tissue outside the vasculature. Image in the right shows higher magnification of inset. ECs, isolectin B4 (green). Scale bar, left, 500 μm, right, 100 μm. ( c ) Haemorrhaging in freshly dissected Itgb1 iECKO P9 brains affecting the cortex, cerebellum, brain stem and the olfactory bulbs. Scale bar, 2 mm. ( d ) Anti-Ter-119 (red) and isolectin B4 (green) immunofluorescence showing strong accumulation of red blood cells around Itgb1 iECKO brain capillaries. Scale bar, 25 μm. ( e ) Sections of P18 control and Itgb1 iECKO brains showing prominent haemorrhaging in mutants. Scale bar, 2 mm. Full size image Arguing further for an important link between integrin β1 and VE-cadherin, many defects seen in Itgb1 iECKO mutants were phenocopied by postnatal, EC-specific inactivation of the Cdh5 gene encoding VE-cadherin ( Supplementary Fig. 8a ). Similarities between the two mutants included the local hyperdensity of the retinal vasculature near the angiogenic front ( Supplementary Fig. 8b ), local haemorrhaging in the peripheral retina ( Supplementary Fig. 8c ), the destabilization of perivenous capillaries in the central vessel plexus ( Supplementary Fig. 8d,e ) and defective sprouting into the deeper retina ( Supplementary Fig. 8f ). In contrast, sprout extension along the vitreous surface of the retina was not visibly impaired in P6 Cdh5 iECKO mutants and, instead, the formation of long sprouts was observed ( Supplementary Fig. 8b ). Thus, most but not all vascular defects seen in Itgb1 iECKO retinas were phenocopied by Cdh5 mutants. The interaction between VE-cadherin and p120 δ -catenin prevents clathrin-dependent endocytosis of the cadherin and is essential for endothelial barrier function [26] , [27] , [28] , [29] . In control retinal vessels, anti-p120 immunosignal was visible at endothelial cell–cell contacts and overlapped with anti-VE-cadherin staining ( Fig. 5a ). In contrast, p120 signals appeared diffuse in Itgb1 iECKO mutants and only weak association with junctions was seen ( Fig. 5a ). In addition, less p120 was bound to VE-cadherin immunoprecipitated from Itgb1 iECKO lung lysates than for littermate controls ( Fig. 5b ). Although VE-cadherin-associated β-catenin was also reduced, no consistent differences were seen for total levels of VE-cadherin, β-catenin and p120 between control and mutant samples ( Fig. 5b ). 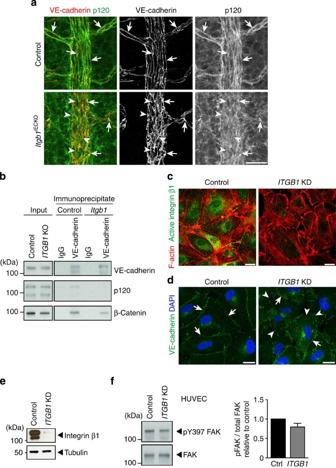Figure 5: Loss of integrin β1 impairs VE-cadherin distribution and p120 association. (a) Maximum intensity projection of anti-VE-cadherin (red) and anti-p120δ-catenin (green) immunostained P18 veins. Double-positive junctional contacts (arrows) can be seen both in controls andthe Itgb1iECKOmutants, but the latter contains VE-cadherin speckles without appreciable p120 association (arrowheads). Scale bar, 30 μm. (b) Western blot analysis of VE-cadherin immunoprecipitated from P18 littermate control and mutant (Itgb1) lung lysates (n=3). Immunoglobulin (IgG) was used as specificity control. Associated p120δ-catenin was reduced inItgb1iECKOsamples compared with controls. A substantial reduction was also seen for β-catenin. Molecular weight marker (kDa) is indicated. (c) The absence of active integrin β1 immunofluorescence (HUTS-4 antibody) in cultured HUVECs afterITGB1KD. F-actin was counterstained with Phalloidin (red). Scale bar, 20 μm. (d) VE-cadherin immunostaining marking cell–cell junctions (arrows) in cultured HUVECs. Cell contact-associated VE-cadherin distribution was discontinuous (arrowheads) afterITGB1KD. Scale bar, 20 μm. (e) Reduced integrin β1 protein expression after siRNA-mediated KD (KD) ofITGB1in cultured HUVECs. (f) Western blot analysis of total and phospho-FAK inITGB1KD or control HUVECs. Molecular weight marker (kDa) is indicated. Right graph shows the relative quantification of signals (n=3, control values set to 1). Figure 5: Loss of integrin β1 impairs VE-cadherin distribution and p120 association. ( a ) Maximum intensity projection of anti-VE-cadherin (red) and anti-p120 δ -catenin (green) immunostained P18 veins. Double-positive junctional contacts (arrows) can be seen both in controls and the Itgb1 iECKO mutants, but the latter contains VE-cadherin speckles without appreciable p120 association (arrowheads). Scale bar, 30 μm. ( b ) Western blot analysis of VE-cadherin immunoprecipitated from P18 littermate control and mutant ( Itgb1 ) lung lysates ( n =3). Immunoglobulin (IgG) was used as specificity control. Associated p120 δ -catenin was reduced in Itgb1 iECKO samples compared with controls. A substantial reduction was also seen for β-catenin. Molecular weight marker (kDa) is indicated. ( c ) The absence of active integrin β1 immunofluorescence (HUTS-4 antibody) in cultured HUVECs after ITGB1 KD. F-actin was counterstained with Phalloidin (red). Scale bar, 20 μm. ( d ) VE-cadherin immunostaining marking cell–cell junctions (arrows) in cultured HUVECs. Cell contact-associated VE-cadherin distribution was discontinuous (arrowheads) after ITGB1 KD. Scale bar, 20 μm. ( e ) Reduced integrin β1 protein expression after siRNA-mediated KD (KD) of ITGB1 in cultured HUVECs. ( f ) Western blot analysis of total and phospho-FAK in ITGB1 KD or control HUVECs. Molecular weight marker (kDa) is indicated. Right graph shows the relative quantification of signals ( n =3, control values set to 1). Full size image Regulation of VE-cadherin internalization To further investigate the link between integrin β1 and VE-cadherin, and exclude potential indirect effects in vivo , we performed small interfering RNA (siRNA) knockdown (KD) experiments in cultured human umbilical cord venous ECs (HUVECs). Successful KD of the human ITGB1 gene was confirmed by immunofluorescence and western blotting, which also revealed reduced activation of FAK ( Fig. 5c–f ). Resembling the situation in the Itgb1 iECKO retinal vasculature, junctional anti-VE-cadherin signals were discontinuous in ITGB1 KD cells and immunostaining was locally weak or absent at cell–cell contacts ( Fig. 5d ). In line with this observation, antibody feeding experiments indicated increased internalization of VE-cadherin in ITGB1 KD HUVECs ( Fig. 6a,b ). The difference between cells transfected with control or ITGB1 siRNAs was enhanced by EGTA-mediated Ca 2+ depletion ( Fig. 6a,b ), a treatment that disrupts Ca 2+ -dependent adhesive interactions between cadherin molecules at cell-cell contact sites [30] . Similar to that in Itgb1 iECKO lung lysates, levels of VE-cadherin protein were unchanged in cultured KD cells ( Figs 5b and 6c ), whereas the association of p120 δ -catenin with immunoprecipitated VE-cadherin was reduced after ITGB1 KD ( Fig. 6c ). Linking these changes to endocytosis, biotinylation experiments indicated accelerated internalization of surface VE-cadherin after ITGB1 KD ( Fig. 6d ). We also investigated the recycling of internalized VE-cadherin back to the cell surface with a reverse biotinylation approach (see Methods). Following EGTA and switch to Ca 2+ -containing medium for 20 or 30 min, a substantial amount of VE-cadherin was back on the cell surface in control but not in ITGB1 KD HUVECs ( Fig. 6e ). Antibody feeding assays also revealed that internalized VE-cadherin was found in early endosome antigen 1-positive early endosomes after ITGB1 KD, which was observed in control cells only after Ca 2+ depletion ( Supplementary Fig. 9a ). Likewise, EGTA-treated control HUVECs showed transient accumulation of VE-cadherin in Rab5-positive endosomes, which did not persist at 15 or 30 min after switching to Ca 2+ -containing medium ( Fig. 6f ). In ITGB1 KD cells, internalized VE-cadherin persisted throughout this time course and was found within and near Rab5-containing vesicular compartments ( Fig. 6f ). Arguing further that matrix signals control endothelial adherens junctions, the association of VE-cadherin and p120 δ -catenin was substantially higher in HUVECs cultured on collagen I or fibronectin than on gelatin ( Supplementary Fig. 9b ). 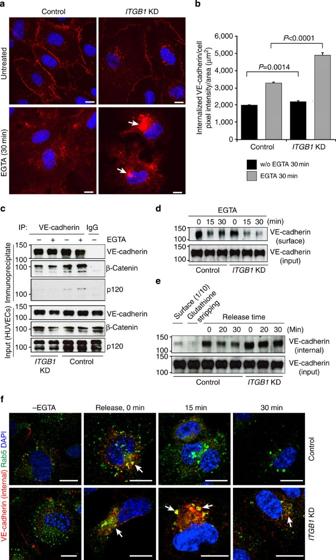Figure 6: Integrin β1 controls VE-cadherin trafficking. (a)ITGB1KD enhanced intracellular (perinuclear) accumulation of antibody-bound VE-cadherin signals (arrows) after EGTA-mediated Ca2+depletion. Scale bar, 10 μm. (b) Analysis of internalized VE-cadherin immunosignals before and after EGTA treatment. Error bars, s.e.m.P-values, one-way analysis of variance. (c) Western blot analysis of p120δ-catenin co-immunoprecipitated with VE-cadherin fromITGB1KD or control HUVECs. Immunoglobulin (IgG) was used as specificity control. Lower panels showing input (lysate) confirm that expression levels of p120 or VE-cadherin were not affected byITGB1KD. (d) Western blotting showing biotinylated (surface) VE-cadherin in cultured HUVECs at the indicated time points after EGTA treatment. Note accelerated internalization of VE-cadherin inITGB1KD HUVECs. Molecular weight marker (kDa) is indicated. (e) Reverse biotinylation assay showing trafficking of VE-cadherin from inside the cell (protected) to the surface (unprotected) following the addition of Ca2+to EGTA-pretreated HUVECs for the indicated times. Note intracellular accumulation of VE-cadherin inITGB1KD cells at 20 and 30 min. Leftmost lane shows aliquot (1/10) of biotinylated (surface) VE-cadherin before EGTA treatment. Efficient removal of coupled biotin was validated by glutathione stripping. (f) Antibody feeding assay showing internal VE-cadherin (red) and partial overlap with Rab5-positive vesicles after release of EGTA-induced Ca2+depletion.ITGB1KD enhanced perinuclear accumulation of VE-cadherin and overlap with Rab5 signal (yellow, arrows) at 15 and 30 min. Nuclei, DAPI (blue). Scale bar, 10 μm. Figure 6: Integrin β1 controls VE-cadherin trafficking. ( a ) ITGB1 KD enhanced intracellular (perinuclear) accumulation of antibody-bound VE-cadherin signals (arrows) after EGTA-mediated Ca 2+ depletion. Scale bar, 10 μm. ( b ) Analysis of internalized VE-cadherin immunosignals before and after EGTA treatment. Error bars, s.e.m. P -values, one-way analysis of variance. ( c ) Western blot analysis of p120 δ -catenin co-immunoprecipitated with VE-cadherin from ITGB1 KD or control HUVECs. Immunoglobulin (IgG) was used as specificity control. Lower panels showing input (lysate) confirm that expression levels of p120 or VE-cadherin were not affected by ITGB1 KD. ( d ) Western blotting showing biotinylated (surface) VE-cadherin in cultured HUVECs at the indicated time points after EGTA treatment. Note accelerated internalization of VE-cadherin in ITGB1 KD HUVECs. Molecular weight marker (kDa) is indicated. ( e ) Reverse biotinylation assay showing trafficking of VE-cadherin from inside the cell (protected) to the surface (unprotected) following the addition of Ca 2+ to EGTA-pretreated HUVECs for the indicated times. Note intracellular accumulation of VE-cadherin in ITGB1 KD cells at 20 and 30 min. Leftmost lane shows aliquot (1/10) of biotinylated (surface) VE-cadherin before EGTA treatment. Efficient removal of coupled biotin was validated by glutathione stripping. ( f ) Antibody feeding assay showing internal VE-cadherin (red) and partial overlap with Rab5-positive vesicles after release of EGTA-induced Ca 2+ depletion. ITGB1 KD enhanced perinuclear accumulation of VE-cadherin and overlap with Rab5 signal (yellow, arrows) at 15 and 30 min. Nuclei, DAPI (blue). Scale bar, 10 μm. Full size image Integrin β1 controls junctional integrity The localization VE-cadherin and its molecular interactions are part of a complex network of upstream and downstream signalling processes [31] , [32] . Although the binding of p120 inhibits VE-cadherin internalization, δ -catenin is also a negative regulator of the Rho/Rho-kinase pathway and myosin light chain (MLC) phosphorylation in ECs [26] , [28] . VE-cadherin promotes Rho-kinase activity, MLC phosphorylation and actomyosin contractility, which, in turn, enhances VE-cadherin accumulation at cell junctions and thereby vessel stability [33] , [34] . The small GTPase Rap1, another important regulator of endothelial junction formation [35] , has been recently shown to promote VE-cadherin-dependent cell–cell adhesion through Cdc42, the kinase MRCK, MLC phosphorylation and actin reorganization [36] . Arguing for a link between integrin β1 and the pathways above, phospho-MLC immunostaining was significantly decreased in the Itgb1 iECKO retinal vasculature ( Fig. 7a ). Moreover, levels of phospho-MLC, as well as active Rap1, Rho and Cdc42 were reduced in ITGB1 KD HUVECs ( Fig. 7b–e ). To elucidate the role of different pathways upstream of phosphorylated MLC, postnatal animals were transiently treated with different pharmacological inhibitors. Blockade of MLC kinase, part of a calcium-dependent pathway controlling phospho-MLC levels, with the inhibitor ML-7 did not lead to haemorrhaging in the retina ( Supplementary Fig. 10a ) and was therefore not investigated further. In contrast, focal bleeding was observed after short-term (4 h) inhibition of MRCK with chelerythrine chloride (CCl) [37] or of Rho-kinase with H-1152 ( Fig. 7f ). Administration of CCl or H-1152 reduced phospho-MLC immunosignals in retinal blood vessels, which was further enhanced by combining the two inhibitors ( Supplementary Fig. 10b ). Single inhibition of MRCK and Rho-kinase also compromised the extension of endothelial sprouts, led to dilation of vessels and disorganization of adherens junctions, and destabilized capillaries in the central retina. Again, these defects were most pronounced after combined treatment with CCl and H-1152 ( Figs 7f and 8a ), indicating that both Rho/Rho-kinase and Rap1/MRCK are acting upstream of p120 δ -catenin in the endothelium. The amount of p120 associated with VE-cadherin immunoprecipitated from mouse lungs was reduced after treatment with CCl or H-1152 and, most efficiently, the combination of the two inhibitors ( Fig. 8b ). In contrast, levels of total VE-cadherin and p120 remained unaltered. Likewise, only the combined siRNA-mediated KD of the Rho-kinases ROCK1/2 and the MRCKs CDC42BPA/CDC42BPB , but not the individual disruption of either pathway, led to a reduced association of p120 δ -catenin and VE-cadherin in HUVECs ( Fig. 8c and Supplementary Fig. 10c ). 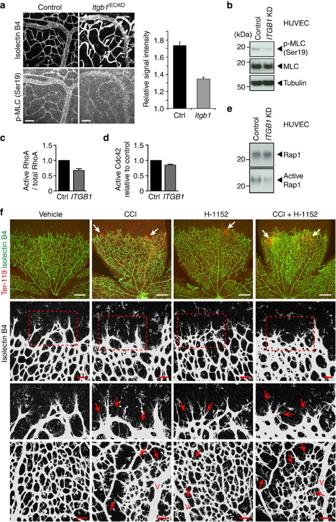Figure 7: Role of actomyosin contractility. (a) Reduced vascular phospho-MLC (Ser19 residue) signals inItgb1iECKOP18 retinas relative to littermate control. Vessels were visualized by isolectin B4 staining. Scale bar, 50 μm. Graph on the right shows quantitation of anti-phospho-MLC immunosignals in P18 control and mutant (Itgb1) retinal veins. Data represents four independent experiments (n=1–3 mice per group each) Error bars, s.e.m.,P<0.001, Student’st-test. (b) Western blot analysis of phospho-MLC (p-MLC) inITGB1KD or control HUVECs (n=3). Molecular weight marker (kDa) is indicated. (c) Active RhoA inITGB1KD or control HUVECs determined by enzyme-linked immunosorbent assay (ELISA). Error bars, s.e.m. (n=3, control values set to 1).P=0.0325, Student’st-test. (d) Active Cdc42 inITGB1KD or control HUVECs determined by ELISA. Error bars, s.e.m. (n=5, control values set to 1).P=0.0079, Student’st-test. (e) Western blot analysis of active Rap1 (Rap1-GTP) inITGB1KD or control HUVECs. Molecular weight marker (kDa) is indicated (n=3). (f) Phenotype of isolectin B4-stained (green/white) P5 wild-type retinas after 4 h of treatment with CCl, H-1152 or both inhibitors, as indicated. Note haemorrhaging (extravasated Ter-119+ erythrocytes, red) in proximity of the angiogenic front (arrows) and altered morphology of sprouts at the angiogenic front of inhibitor-treated animals (images in second row). Higher magnification images of insets (row 3) show defective extension of sprouts but the presence of filopoda (red arrows). Inhibitors also triggered destabilization of capillaries around arteries and veins (V) in the central plexus, as indicated by high abundance of thin endothelial connections (red arrows in row 4). Scale bar, row 1, 200 μm, row 2, 20 μm, row 4, 50 μm. Data represents three repetitions (n=3-4 pups per group each). Figure 7: Role of actomyosin contractility. ( a ) Reduced vascular phospho-MLC (Ser19 residue) signals in Itgb1 iECKO P18 retinas relative to littermate control. Vessels were visualized by isolectin B4 staining. Scale bar, 50 μm. Graph on the right shows quantitation of anti-phospho-MLC immunosignals in P18 control and mutant ( Itgb1 ) retinal veins. Data represents four independent experiments ( n =1–3 mice per group each) Error bars, s.e.m., P <0.001, Student’s t -test. ( b ) Western blot analysis of phospho-MLC (p-MLC) in ITGB1 KD or control HUVECs ( n =3). Molecular weight marker (kDa) is indicated. ( c ) Active RhoA in ITGB1 KD or control HUVECs determined by enzyme-linked immunosorbent assay (ELISA). Error bars, s.e.m. ( n =3, control values set to 1). P =0.0325, Student’s t -test. ( d ) Active Cdc42 in ITGB1 KD or control HUVECs determined by ELISA. Error bars, s.e.m. ( n =5, control values set to 1). P =0.0079, Student’s t -test. ( e ) Western blot analysis of active Rap1 (Rap1-GTP) in ITGB1 KD or control HUVECs. Molecular weight marker (kDa) is indicated ( n =3). ( f ) Phenotype of isolectin B4-stained (green/white) P5 wild-type retinas after 4 h of treatment with CCl, H-1152 or both inhibitors, as indicated. Note haemorrhaging (extravasated Ter-119+ erythrocytes, red) in proximity of the angiogenic front (arrows) and altered morphology of sprouts at the angiogenic front of inhibitor-treated animals (images in second row). Higher magnification images of insets (row 3) show defective extension of sprouts but the presence of filopoda (red arrows). Inhibitors also triggered destabilization of capillaries around arteries and veins (V) in the central plexus, as indicated by high abundance of thin endothelial connections (red arrows in row 4). Scale bar, row 1, 200 μm, row 2, 20 μm, row 4, 50 μm. Data represents three repetitions ( n =3-4 pups per group each). 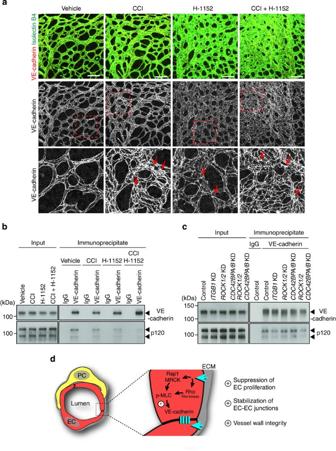Figure 8: Actomyosin contractility controls endothelial junctions. (a) Morphology of isolectin B4 (green)- and anti-VE-cadherin (red/white)-stained vessels in the perivenous plexus of P10 wild-type retinas treated with the indicated inhibitors. CCl, H-1152 or the combination of both led to vessel dilation and disorganization of VE-cadherin at cell–cell junctions (red arrows). Images in row 3 show higher magnifications of insets in the second row. Scale bar, 50 μm. Data represents three repetitions (n=3–4 pups per group each). (b) Western blot analysis of VE-cadherin immunoprecipitated from lung lysates of inhibitor-treated or vehicle control P10 mice (n=3). Note reduced association of p120 with VE-cadherin after inhibitor treatmentin vivo. Immunoglobulin (IgG) was used as specificity control. Levels of total p120 or VE-cadherin in lung lysates were not altered by inhibitors, as by shown panels on the left (input). Molecular weight marker (kDa) is indicated. (c) Western blot analysis (n=3) of p120δ-catenin co-immunoprecipitated with VE-cadherin from control HUVEC or after KD ofITGB1,ROCK1/2,CDC42BPA/B(the genes encoding MRCKα and MRCKβ), or combined KD ofROCK1/2andCDC42BPA/B. Immunoglobulin (IgG) was used as specificity control. Left panels showing input (lysate) confirmed equal expression of p120 or VE-cadherin. (d) Schematic summary of findings. Endothelial integrin β1 suppresses endothelial proliferation and stabilizes cell junctions by regulating the trafficking of VE-cadherin. Integrin β1 controls phospho-MLC (p-MLC) levels, endothelial actomyosin contractility and thereby VE-cadherin localization at cell–cell contacts through the Rap1/MRCK and Rho/Rho-kinase pathways, which have partially redundant roles in the regulation of vessel wall integrity. Full size image Figure 8: Actomyosin contractility controls endothelial junctions. ( a ) Morphology of isolectin B4 (green)- and anti-VE-cadherin (red/white)-stained vessels in the perivenous plexus of P10 wild-type retinas treated with the indicated inhibitors. CCl, H-1152 or the combination of both led to vessel dilation and disorganization of VE-cadherin at cell–cell junctions (red arrows). Images in row 3 show higher magnifications of insets in the second row. Scale bar, 50 μm. Data represents three repetitions ( n =3–4 pups per group each). ( b ) Western blot analysis of VE-cadherin immunoprecipitated from lung lysates of inhibitor-treated or vehicle control P10 mice ( n =3). Note reduced association of p120 with VE-cadherin after inhibitor treatment in vivo . Immunoglobulin (IgG) was used as specificity control. Levels of total p120 or VE-cadherin in lung lysates were not altered by inhibitors, as by shown panels on the left (input). Molecular weight marker (kDa) is indicated. ( c ) Western blot analysis ( n =3) of p120 δ -catenin co-immunoprecipitated with VE-cadherin from control HUVEC or after KD of ITGB1 , ROCK1/2 , CDC42BPA/B (the genes encoding MRCKα and MRCKβ), or combined KD of ROCK1/2 and CDC42BPA/B . Immunoglobulin (IgG) was used as specificity control. Left panels showing input (lysate) confirmed equal expression of p120 or VE-cadherin. ( d ) Schematic summary of findings. Endothelial integrin β1 suppresses endothelial proliferation and stabilizes cell junctions by regulating the trafficking of VE-cadherin. Integrin β1 controls phospho-MLC (p-MLC) levels, endothelial actomyosin contractility and thereby VE-cadherin localization at cell–cell contacts through the Rap1/MRCK and Rho/Rho-kinase pathways, which have partially redundant roles in the regulation of vessel wall integrity. Full size image Taken together, these data argue that integrin complexes involving the β1-subunit are indispensable for the formation of stable, mature and non-leaky vessels. The molecular processes downstream of integrins involve MLC phosphorylation through Rap1 and the kinase MRCK, as well as Rho/Rho-kinase signalling ( Fig. 8d ). The sum of our work establishes several novel roles of integrin β1 in vessel growth and stabilization ( Fig. 8d ). These data also demonstrate that the β1-subunit has critical context-dependent functions. Although the integrin is required for the extension of endothelial sprouts at the angiogenic growth front, it also suppresses classical angiogenic activities such as sprouting and EC proliferation in the perivenous vessel plexus. The Itgb1 iECKO phenotype in the present study differs substantially from what was reported for an independently generated, inducible Itgb1 mutant, which only displayed defects in a fraction of arterial ECs [15] . This may reflect differences in the efficiency of Cre transgenics [38] , [39] and of conditional Itgb1 strains [16] , [40] . The whole open reading frame of the Itgb1 gene is flanked by loxP sites in the line employed for most of the experiments by Zovein et al . [15] and, as was shown by the same group, integrin β1 protein expression in this mouse strain can persist from a circular DNA fragment even after Cre recombination [41] . Delayed loss of protein expression was not an issue in our experiments and, instead, we observed rapid formation of vascular defects and limited survival of Itgb1 iECKO mutants after tamoxifen administration ( Supplementary Fig. 3a ). Although we also did not observe previously reported arterial malformations [15] , this might be a consequence of limited mutant survival and severe defects in Itgb1 iECKO veins and capillaries. Another important question concerns the identity of the integrin α-subunits and matrix molecules that interact with integrin β1 in the vasculature. The matrix protein laminin α4 regulates tip cell number and vessel density in the retina, which involves different endothelial integrin receptors [42] . Vascular defects have been also reported in the original publication of the Lama4 gene knockout [43] . However, the survival of these global and constitutive mutants is distinct from the lethality of Itgb1 iECKO mice, suggesting involvement of other matrix molecules. Fibronectin binding to α5β1 heterodimers mediates the adhesion of endothelial filopodia to astrocytic matrix [44] . EC-specific targeting of the α5 and αv integrins, the major fibronectin receptors in the endothelium, led to the formation of oedema but did not substantially impair angiogenesis in the embryo [45] . Inactivation of Itga3 or Itga4 , the genes encoding the α3- and α4-subunits, respectively, in ECs was also compatible with mutant survival [46] , [47] . This argues for contributions of multiple α-subunits, which control EC behaviour together with integrin β1 in response to matrix signals or other, as yet unidentified, cues. The combination of inducible, cell type-specific mouse genetics and high-resolution imaging in the retinal vasculature has allowed us to gain deeper insight into the biological function of β1-containing integrins and led to the discovery of a novel role involving VE-cadherin stabilization at endothelial junctions. Previous work on other members of the cadherin family, in most cases E-cadherin, has shown that these adhesion molecules can control integrin activity [48] , [49] . At the molecular level, this has been linked to the small GTPase Rap1, a mediator of integrin inside-out activation [10] , [50] . Rap1 can also promote cell junction formation [48] , [51] and, according to our data, might mediate bidirectional cross-talk between cadherins and integrins in ECs. Rap1 and the kinase MRCK, as well as Rho/Rho-kinase, appear to act redundantly in the control of actomyosin contractility downstream of integrins. This promotes binding of p120 δ -catenin to VE-cadherin and stabilizes adherens junctions. Nevertheless, given the great complexity of signalling interactions involving integrins and cadherins, other pathways may also contribute to the junction defects seen in the Itgb1 iECKO vasculature. The great importance of endothelial junctions in many pathobiological processes involving enhanced vascular permeability is well recognized and there is increasing evidence for critical roles of VE-cadherin internalization [52] , [53] , [54] . Thus, changes affecting ECM composition or enhanced ECM degradation by metalloproteinases, as observed in stroke, age-related macular degeneration, diabetic retinopathy, chronic inflammation or other human diseases [55] , [56] , [57] , [58] , may affect endothelial integrin activity and thereby contribute to endothelial barrier breakdown. Our findings now clearly indicate that alterations in integrin activity can affect the sealing of endothelial cell–cell contacts. As it might be difficult to suppress ECM degradation and remodelling in acute or chronic pathologies, understanding of the molecular pathways linking integrin signalling to VE-cadherin function might be useful for the development of strategies preventing endothelial barrier breakdown in human disease. Mutant mice and inducible genetic experiments Pdgfb-iCre transgenics [17] were bred into a background of Itgb1 (ref. 16 ) or Cdh5 (ref. 24 ) conditional (loxP-flanked) mice. To induce Cre activity, newborn offspring from a Pdgfb-iCre Itgb1 lox/+ × Itgb1 lox/lox intercross were given intraperitoneal tamoxifen injections of 50 μl (Sigma, T5648; 1 mg ml −1 in ethanol/peanut oil) on P2–3, P3–7 or P10–13, respectively. The phenotypes of Pdgfb-iCre × Itgb1 lox/lox ( Itgb1 iECKO ) mutants were analysed at postnatal stages P6, P9 or P18, respectively. For Cdh5 , three intraperitoneal tamoxifen injections were given at P1–3 and phenotypes were analysed at P6 or P9. In all genetic experiments, tamoxifen-injected littermate animals were used as control, and both male and female animals were used. For the pharmacological inhibition of Rho-kinase and MRCK signalling in vivo , we intraperitoneally injected the indicated combinations of vehicle, the MLCK inhibitor ML-7 (Sigma; 133.3 mg kg −1 ), the Rho-kinase inhibitor H-1152 (Merck Millipore; 26.7 mg kg −1 ) or the MRCK inhibitor CCl [37] (Merck Millipore; 10 mg kg −1 ). Retinas and lungs were collected 4 h after injection at P5 or P10, as indicated. Immunostainings were performed in triplicate, unless indicated otherwise. All animal experiments were performed in compliance with the relevant laws and institutional guidelines, were approved by local animal ethics committees and were conducted with permissions granted by the Landesamt für Natur, Umwelt und Verbraucherschutz (LANUV) of North Rhine-Westphalia. Immunohistochemistry and EdU labelling All immunostainings were carried out with littermate tissues processed simultaneously under the same conditions, as described previously [59] , [60] . In brief, to analyse (and quantitate) the morphology of the retinal vasculature and preserve intact endothelial filopodia and sprouts at the angiogenic front, whole animal eyes were fixed in 4% paraformaldehyde (PFA) at 4 °C overnight. The following day, the eyes were washed in PBS before retinas were dissected and partially cut in four quadrants. After blocking/permeabilization in 1% BSA with 0.3% Triton X-100 for several hours at room temperature or overnight at 4 °C, the retinas were washed two times in Pblec buffer (1% Triton X-100, 1 mM CaCl 2 , 1 mM MgCl 2 and 0,1 mM MnCl 2 in PBS pH 6.8) for 20 min and incubated for overnight in Pblec containing biotinylated isolectin B4 (1:50, VectorLabs). Following five washes (each 20 min) in blocking solution, retinas were incubated with Alexa Fluor streptavidin-conjugated antibodies (Life Technologies, 1:100) for 2 h, washed three times more and flat-mounted in microscope glass slides with Fluoromount-G (SouthernBiotech, 0100-01). Double or triple whole-mount immunohistochemistry was performed in retinas fixed 2 h on ice in 4% PFA or in MeOH at −20 °C. After fixation, retinas were blocked for 2 h in 1% BSA with 0.3% Triton X-100 and incubated overnight or for 2 h with isolectin B4 (Vector Labs, 1:50) and the following primary antibodies: rat anti-VE-cadherin (BD Biosciences, 1:200), rat anti-Integrin β1 (Chemicon, 1:200), rabbit anti-laminin α4 (serum 377, 1:1,000) [61] , rabbit anti-Collagen IV (Serotec, 1:200), rabbit anti-fibronectin (Sigma, 1:200), rat anti-ICAM2 (BD Biosciences, 1:200), rabbit anti-Claudin5 (Life Technologies, 1:200), rabbit anti-p120 (Santa Cruz, 1:200), rat anti-active integrin β1 (9EG7; BD Biosciences, 1:200), rat anti-Ter119 (R&D Systems, 1:200), goat anti-ESM1 (R&D, 1:200), anti-α-smooth muscle actin-Cy3 (Sigma, 1:100), goat anti-CD31 (R&D, 1:100) and rabbit anti-phospho-MLC 2 (Ser19) (Cell Signaling, 1:100). For detection, suitable species-specific Alexa Fluor-coupled secondary antibodies (1:500) were used. For labelling of proliferating cells, 100 μg of EdU (Life Technologies) per pup was injected intraperitoneally 4 h before killing. Following isolectin B4 staining, retinas were isolated and processed as described before [60] . EdU-positive cells were detected with the Click-iT EdU Alexa Fluor-647 Imaging Kit (Life Technologies, C10340). Morphological and histological analysis of adult brain Terminally anaesthetized animals were perfused intracardially with PBS, followed by PBS containing 4% PFA. Whole brains, dissected from P9 or P18 mice, were photographed using a charge-coupled device camera mounted on a dissecting microscope. Brains were then submerged in 4% PFA in PBS overnight at 4 °C before they were cut on a vibratome in 100-μm-thick sections and stained with isolectin B4 (1:50) and rat anti-Ter119 antibody (R&D Systems, 1:400). Suitable species-specific Alexa Fluor-coupled secondary antibodies (1:500) were used. Western blotting and immunoprecipitation For the analysis of protein levels in mutant mouse pups, postnatal lungs were dissected out, transferred to a reagent tube and frozen in liquid nitrogen. On the day of western blot analysis, the tissue was lysed in PL buffer (20 mM Tris-HCl pH 8.0, 1 mM EDTA, 1 mM dithiothreitol, phosphatase inhibitor cocktail SetV (Calbiochem, 524629), 1 mM Na 3 VO 4 , protease inhibitor cocktail (Sigma, P2714, 1:10), 1% TritonX-100, 150 mM NaCl) and homogenized with a cylindrical glass and pestle (Potter-Elvehjem). Tissue debris was removed by centrifugation and the supernatant was diluted in loading buffer and analysed by SDS–PAGE and western blotting. See Supplementary Fig. 11 for full scans of western blottings. Blots were quantified with the gel analysis function in the programme ImageJ. The following antibodies were used for immunoblotting: rabbit anti-actin (Sigma, 1:4,000), rat anti-Endomucin (clone V.7C7, Santa Cruz, 1:4,000), rabbit anti-p120 (Santa Cruz, 1:1,000), goat anti-β-catenin (R&D Systems, 1:1,000), rabbit anti-cyclin D1 (Cell Signaling, 1:1,000), rabbit anti-cyclin A1 (Santa Cruz, 1:1,000), rabbit anti-p27Kip1 (Cell Signaling, 1:1,000), goat anti-VE-cadherin (Santa Cruz, 1:1,000), rat anti-VE-cadherin (BD Biosciences, 1:500), rabbit anti-VE-cadherin (Cell Signaling, 1:1,000), rabbit anti-integrin β1 (Chemicon, 1:1,000), rabbit anti-ROCK1 (Abcam, 1:500), rabbit anti-ROCK2 (Cell Signaling, 1:500), rabbit anti-CDC42 binding protein kinase-α (Abcam, 1:500), mouse anti-CDC42BPB (AbD Serotec, 1:500), rabbit anti-FAK (Cell Signaling, 1:1,000), rabbit anti-phospho-FAK(Tyr397) (Cell Signaling, 1:1,000), mouse anti-β-catenin (BD Biosciences, 1:1,000), rabbit anti-phospho-MLC2 (Ser19) (Cell Signaling, 1:100), mouse anti-MLC (Sigma, 1:500) and mouse anti-tubulin (Sigma, 1:5,000). For immunoprecipitation of VE-cadherin from lung lysates, mouse lungs were homogenized in lysis buffer (20 mM Tris-HCl pH 8.0, 1 mM EDTA, 150 mM NaCl, 0.5% Triton X-100, 0.5% NP-40, PhosSTOP (Roche)), protease inhibitor cocktail (Sigma, P2714) and clarified by centrifugation at 20,000 g for 30 min at 4 °C. The soluble supernatants were incubated with protein G sepharose beads with VE-cadherin antibody (Santa Cruz; 2 μg) for 1 h at 4 °C, washed three times with lysis buffer and finally dissolved by boiling in SDS–PAGE sample buffer. For immunoprecipitation of VE-cadherin from cell lysates, cells were homogenized in lysis buffer (20 mM Tris-HCl pH 7.5, 150 mM NaCl, 0.5% NP-40, PhosSTOP, protease inhibitor cocktail) and clarified by centrifugation at 20,000 g for 20 min at 4 °C. After examining the total protein concentration of lysates by Precision Red Advanced protein assay reagent (Cytoskeleton), the soluble supernatants were incubated with protein G sepharose beads with VE-cadherin antibody (Santa Cruz; 2 μg) for 2 h at 4 °C, washed three times with lysis buffer and finally dissolved by boiling in SDS–PAGE sample buffer. Immunoblot analysis was performed with the indicated antibody as described above. GTP-Rap1 pull-down assay The activity of Rap1 was determined by pull-down assay with Rap1 Activation Kit (Merck Millipore), according to the manufacturer’s instructions. In brief, the cells were washed with ice-cold PBS and lysed in lysis buffer (50 mM Tris-HCl, pH 7.5, 1 mM EGTA, 10 mM MgCl 2 , 500 mM NaCl, 0.5% NP-40, protease inhibitor cocktail). The lysates were centrifuged at 20,000 g for 10 min at 4 °C and the supernatants were incubated with beads conjugated 20 μg of GST-Ral-GDS-RBD for 30 min at 4 °C. The beads were washed with an excess of lysis buffer and then eluted with SDS–PAGE sample buffer. The eluates were subjected to SDS–PAGE, followed by immunoblot analysis with the rabbit anti-Rap1 antibody (Merck Millipore, 07-916, 1:500). Measurement of active and total RhoA and Cdc42 Active and total RhoA were measured by RhoA G-LISA Activation Assay and Total RhoA ELISA (Cytoskeleton) by using 1.2 mg per ml protein per sample, according to the manufacturer’s instructions. In brief, the cells were washed with ice-cold PBS, lysed in provided lysis buffer, centrifuged and snap frozen in liquid nitrogen. After examining the total protein concentration of lysates by Precision Red Advanced protein assay reagent, adjusted supernatants were applied into assay plates, incubated with primary antibody, secondary antibody, followed by the incubation with detection reagent. The plates were read by a Synergy 2 multi-mode plate reader (OD 490 nm; BioTek). Data were processed as a ratio of active RhoA/total RhoA; the control values of the control group were set to 1. Active Cdc42 was measured by Cdc42 G-LISA Activation Assay (Cytoskeleton) by using 0.5 mg per ml protein per sample, according to the manufacturer’s instructions. In brief, the cells were washed with ice-cold PBS, lysed in provided lysis buffer, centrifuged and snap frozen in liquid nitrogen. After examining the total protein concentration of lysates by Precision Red Advanced protein assay reagent, adjusted supernatants were applied into assay plates, incubated with primary antibody, secondary antibody, followed by the incubation with detection reagent. The plates were read by a Synergy 2 multi-mode plate reader (OD 490 nm). The control values of the control group were set to 1. Quantitative RT–PCR analysis Total RNA was isolated from lung with RNeasy Mini Kit (QIAGEN) and 500 ng per reactin was used to generate complementary DNA with iScript cDNA Synthesis Kit (BIO-RAD). Quantitative PCR was performed by using an ABI PRISM 7900HT Fast Real-Time PCR System (Life Technologies). TaqMan gene expression assays for murine Actb (4352341E), Cdh5 (Mm00486938_m1), Kdr (Mm01222419_m1), Flt4 (Mm01292608_m1), Dll4 (Mm01292608_m1), Notch1 (Mm00435245_m1), Mmp1a (Mm00473485_m1), Mmp2 (Mm00439498_m1), Mmp9 (Mm00442991_m1) and Mmp14 (Mm00485054_m1) were used in combination with TaqMan Gene Expression Master Mix (Life Technologies). Gene expression was normalized to the endogenous control Actb . The relative expression differences obtained represent the average of the results obtained for two independent animals per group from two independent litters with duplicate reactions for each gene. Endothelial cell culture and siRNA KD experiments HUVEC cells purchased from Life Technologies were maintained in Medium200 (M200) supplemented with low serum growth supplement (Life Technologies). HUVEC cells at passage 3–6 were used for experiments. HUVEC cells seeded on 0.2% Gelatin (Sigma), 5 μg ml −1 fibronectin (Sigma) or 500 μg ml −1 collagen I (BD Biosciences) coated dishes were transfected with siRNAs by using oligofectamine (Life Technologies) according to the manufacturer’s instructions. The following target sequences were used: human ITGB1 #6 (5′- GGTAGAAAGTCGGGACAAA -3′) and #7 (5′- TGATAGATCCAATGGCTTA -3′) (Thermo Fisher Scientific Inc.), human ROCK1 s12098 (5′- CGGTTAGAACAAGAGGTAA -3′), s12099 (5′- GCTTGTAGGTGATACACCT -3′), human ROCK2 s18161 (5′- GGAGATTACCTTACGGAAA -3′), s18162 (5′- GAGATTACCTTACGGAAAA -3′), human CDC42BPA s16096 (5′- CCGCAATCATAGATCATGA -3′), s16098 (5′- GATGGAAGATGGAACGGTT -3′), human CDC42BPB s18401 (5′- CGAGAACGGCATAACGAGA -3′), s18402 (5′- CACTCAACTCCATCGAATA -3′) (Life Technologies). ON-TARGETplus negative control siRNA (Thermo Fisher Scientific Inc.) Silencer Negative Control No.1 siRNA (Life Technologies) were used for control transfections. Efficiency of KD was evaluated by western blotting or immunofluorescence staining. Experiments were started 48 or 72 h after transfection. After treatment, HUVEC cells were fixed in 4% PFA in PBS at 4 °C for 30 min, before they were incubated with NH 4 Cl for 10 min at room temperature and blocked with PBS containing 3% BSA (Sigma) for 1 h at room temperature. Next, cells were permeabilized using 0.2% Triton X-100 in PBS at room temperature for 5 min and quenched for 10 min with NaBH 4 (0.5 mg ml −1 in PBS; Sigma). Cells were incubated with primary antibody for 1 h at room temperature, washed three times with PBS and incubated with appropriate secondary antibodies for 1 h at room temperature. Concentrations of primary antibodies used were as follows: mouse anti-human active integrin β1 (HUTS-4, Chemicon, 1:100), goat anti-VE-cadherin (Santa Cruz, 1:100) and rabbit anti-Rab5 (Cell Signaling, 1:100). Actin was visualized using Alexa Fluor 546-conjugated phalloidin (Life Technologies, 1:400). Nuclei were stained using DAPI (Sigma, D9542) before cells were embedded in mounting media. Ca 2+ switch experiments were performed using a well-established protocol [62] . Briefly, HUVEC monolayers were incubated in medium supplemented with 4 mM EGTA for 30 min at 37 °C to disrupt VE-cadherin-mediated interactions. Treated cells were then either lysed or allowed to reform junctions by further incubation in fresh medium containing 1.8 mM Ca 2+ for the indicated times at 37 °C. Internalization and recycling experiments For surface biotinylation assays, the cells of 10-cm dish were incubated at 37 °C for the indicated time, to allow internalization in 4 mM EGTA in M200, were then chased in the same medium for the indicated periods of time. At the end of the chase, the cells were washed with ice-cold PBS containing 0.1 mM CaCl 2 and 1 mM MgCl 2 (PBS+). Next, plates were incubated at 4 °C with 4 ml of 0.5 mg ml −1 sulfo-NHS-biotin (Thermo Fisher Scientific) in PBS+ for 1 h. The reaction was stopped by washing with ice-cold glycine solution (100 mM glycine, pH 7.5) before cells were lysed in lysis buffer (1% NP-40, 1% Triton X-100, 50 mM Tris-HCl pH 8.0, 150 mM NaCl, protease inhibitor cocktail (Sigma) and phosphatase inhibitor cocktail Set V (Calbiochem)). Biotinylated proteins were precipitated by streptavidin-agarose (Life Technologies) and analysed by western blotting. For reverse biotinylation experiments, cells were incubated at 4 °C with 4 ml of 0.5 mg ml −1 sulfo-NHS-SS-biotin (Thermo Fisher Scientific) for 1 h. After washing with ice-cold glycine solution, cells were incubated at 37 °C for 30 min to allow internalization in 4 mM EGTA in M200. After washing, cells were allowed to recover in complete calcium-containing culture medium for the indicated time and were then washed three times with ice-cold PBS+ on ice. Samples were incubated twice for 20 min with 45 mM of the membrane-non-permeable reducing agent glutathione S -transferase in 75 mM NaCl, with 75 mM NaOH and 1% FCS added just before use (stripping buffer). Cells were further washed twice on ice with PBS+ and incubated for 30 min with iodoacetamide (in PBS+ with 1% FCS; quenching buffer) to quench free sulfo-reactive groups. To evaluate total labelling of surface, a sample for control cells was not stripped with glutathione S -transferase. Then, cells were lysed in lysis buffer. To evaluate background labelling of the stripping, one control sample was stripped without incubation at 37 °C. Biotinylated proteins were then precipitated by streptavidin-agarose and analysed by western blotting. Antibody feeding experiments Before transfection, HUVEC cells were cultured on gelatin-coated (0.2%, 37 °C for 30 min) cover slips in M200 medium. After 24 h, the cells were transfected with the intended siRNA using oligofectamine, according to the manufacturer’s instructions. After 48 h, HUVEC cells were incubated with the anti-VE-cadherin antibody (Abcam, diluted 1:40 in culture medium) for 30 min at 37 °C. Cells were rinsed with PBS+ and transiently exposed to 4 mM EGTA for 30 min to disrupt Ca 2+ -dependent intercellular junctions. After washing, cells were allowed to recover in complete cell calcium-containing culture media for the indicated time. After rinsing with PBS+ on ice, cells were fixed with 4% PFA for 30 min on ice and blocked with 1% BSA for 10 min at room temperature. Following incubation with an excess amount of anti-mouse IgG Alexa 633-conjugated antibody (Life Technologies, 1:100) for 1 h to block any antibody remaining on the cell surface, cells were rinsed with PBS+ 3 times and permeabilized with 0.2% Triton X-100. Endocytosed VE-cadherin was visualized with anti-mouse IgG Alexa 546-conjugated antibody (Life Technologies, 1:400) and imaged with an SP5 confocal microscope (Leica). To quantify VE-cadherin internalization, the total fluorescent intensity within a cell was measured and divided by its area (sum of pixel intensity/μm 2 ). The data represent the mean and the s.e.m. of more than 30 cells in each condition. All images were acquired under identical parameters. The data are representative of three independent experiments. Quantitative analysis of the retinal vasculature All quantifications were done on high-resolution confocal images representing a thin z section of the sample. The number of branchpoints and the area covered by ECs were calculated with the Volocity (Perkin Elmer) software from 24 fields sized 770 × 770 μm, 6 retina samples per group. The number of endothelial sprouts and filopodial extensions were quantified at the angiogenic front in 24 fields (sized 385 × 385 μm, 6 retinas per group) of control ( Itgb1 lox/lox) and Itgb1 iECKO retinas. The total number of filopodia was normalized for a standard size (100 μm in length) of vessels at the angiogenic front. EdU-labelled isolectin B4-positive ECs were counted in 16 fields (sized 385 × 385 μm, 4 retinas per group). Vascular progression was measured by defining a straight line from the angiogenic front to the centre of the retina for each retina quadrant. A minimum of 16 quadrants belonging to 4 retinas per group were used for quantification. Intensity of laminin α4, collagenIV, fibronectin, pMLC staining which was positive for isolectin B4 staining was measured with the Volocity. Data are based on a minimum of three independent experiments or three mutant and control animals for each stage and result shown. Electron microscopy For electron microscopy, mouse retinas were chemically fixed and embedded in epon following a protocol published by Möbius et al . [63] In brief, terminally anaesthetized mice were perfused with 10 ml PBS followed by 40 ml fixative (2% glutaraldehayde, 2% PFA in 0.2 M cacodylate buffer, pH 7.2). Eyes were removed and directly dissected in fixative so that retinas were flattened into four sections. Sample were post-fixed with 1% osmiumtetroxide and embedded in epon. In a distance of 300 μm from the outer edge of flattened retinas, 60 nm ultrathin sections were collected (UC6, Leica, Vienna, Austria), counterstained by uranyl and lead, and examined at the electron microscope (Tecani12-biotwin, FEI, Eindhoven, the Netherlands). Vessels images were recorded with a megaview charge-coupled device camera (SIS-Olympus, Münster, Germany) and high-resolution pictures with Ditabis plates (Ditabis, Pforzheim, Germany). Image acquisition and processing Stained and flat mounted retinas were analysed at high resolution with Leica TCS SP5 and TCS SP8 confocal microscopes, a Zeiss LSM 780 confocal microscope (Zeiss) or, at lower resolution, with a Leica Stereomicroscope MZ16F coupled to a digital camera (Hamamatsu C4742-95). Volocity, Photoshop CS and Illustrator CS (Adobe) software were used for image acquisition and processing. All images shown where immunostaining levels are compared are representative of at least six different images from three different retina immunostainings per group where the laser excitation and confocal scanner detection settings were the same. How to cite this article: Yamamoto, H. et al . Integrin β1 controls VE-cadherin localization and blood vessel stability. Nat. Commun. 6:6429 doi: 10.1038/ncomms7429 (2015).